Ultra-flexible solution-processed organic field-effect transistors Organic semiconductors might enable new applications in low-cost, light-weight, flexible electronics. To build a solid foundation for these technologies, more fundamental studies of electro-mechanical properties of various types of organic semiconductors are necessary. Here we perform basic studies of charge transport in highly crystalline solution-processed organic semiconductors as a function of applied mechanical strain. As a test bed, we use small molecules crystallized on thin plastic sheets, resulting in high-performance flexible field-effect transistors. These devices can be bent multiple times without degradation to a radius as small as ~200 μm, demonstrating that crystalline solution-processed organic semiconductors are intrinsically highly flexible. This study of electro-mechanical properties suggests that solution-processable organic semiconductors are suitable for applications in flexible electronics, provided that integration with other important technological advances, such as device scalability and low-voltage operation, is achieved in the future. Organic electronics is an emerging technology with a promise in applications where very high-performance semiconductor devices are not necessary. These applications include disposable electronics, smart cards, light-emitting diodes, signage, wearable electronics and sensors [1] . To make organic electronics competitive with inorganic semiconductors for these niche applications, the fabrication techniques should rely on very simple and inexpensive approaches, such as solution deposition of organic semiconductors on plastic substrates, in which the fabrication process should ideally be performed in air and at room temperature. In addition, to compete with flexible forms of inorganic semiconductors, such as ultra-thin single-crystal silicon (see, for example, a review by Rogers and colleagues [2] ), these organic circuits must also exhibit a very good electro-mechanical stability, that is, mechanical flexibility without degradation of the electrical performance. Provided that low-cost fabrication on plastic sheets and mechanical flexibility are truly realized, organic electronics might enable new applications exploiting the unique properties of carbon-based materials. Although organic semiconductors have been long envisioned as materials suitable for flexible electronics, an overwhelming majority of studies in this field, especially those dealing with organic field-effect transistors (OFETs), are still performed using rigid substrates, such as glass or expensive Si/SiO 2 wafers. Such an approach can be justified for basic research, but it does not address the agenda of low-cost, flexible electronics. Therefore, more basic studies of mechanical stability and the impact of strain on fundamental electronic properties of organic semiconductors on flexible platforms are necessary. The effort on incorporating flexible/stretchable plastic substrates and gate insulators in organic electronic devices is still very young (for reviews, see the MRS Bulletin themed issue on ‘Materials for stretchable electronics’) [3] . Within this effort, there are a few papers that perform tests of mechanical flexibility of organic devices and investigate the dependence of their performance on mechanical strain. For example, Briseno et al . [4] developed high-performance flexible single-crystal rubrene OFETs on Kapton substrates with a field-effect mobility μ ~5 cm 2 V −1 s −1 that could be bent to a radius of R ~6 mm without degradation. Sekitani et al . [5] made an important next step toward more practical devices and demonstrated vacuum-evaporated pentacene OFETs supported by polyimide substrates with mobility μ ~0.5 cm 2 V −1 s −1 that could be bent to a radius of R ~3.5 mm (for devices without encapsulation) and down to 100 μm (for devices encapsulated in parylene). Comparable results were obtained by Sokolov et al . [6] using small molecules evaporated on polymer dielectrics in high vacuum. Uno et al . [7] also used high-vacuum evaporation of an organic semiconductor on flexible substrates using parylene as a gate insulator to achieve vertical OFETs with μ =0.15–0.2 cm 2 V −1 s −1 [6] ). The key advantage of their transistor design was an interdigitated three-dimensional structure, allowing for a high output current, but mechanical flexibility was moderate, with the smallest bending radius of ~7 mm. Finally, Smith et al . [8] combined a solution-processed small-molecule organic semiconductor with a polymeric gate insulator in a top-gated OFET configuration on plastic substrates. However, the data on mechanical flexibility of these devices are unavailable. In addition, conjugated polymer OFETs on plastic substrates have been demonstrated by Yan et al . and Cho et al . [9] , [10] However, these studies did not address the mechanical properties of the devices either. It’s important to emphasize that the few works above are mentioned here only as representative examples in this area (for a comprehensive review, see ref. 3 ). These initial studies of OFETs on plastics and a few reports on their mechanical robustness are very encouraging. Nevertheless, there is clearly a lack of rigorous basic tests of mechanical flexibility of various types of organic semiconductors and especially those based on solution-processed small molecules. The latter class of materials yields highly crystalline (moderately high mobility) thin films deposited from solutions and is thus very promising for development of low-cost printed electronics. To address the fundamental question of how the electrical properties of these materials respond to mechanical flexing, we focused our attention on measurements of charge carrier mobility in two representative solution-crystallized organic semiconductors as a function of strain applied in various experimental configurations (at varied bending radius, bending angle, number of bending cycles, under compressive and tensile strain). Our results indicate that these crystalline semiconducting films are intrinsically highly flexible, with devices still operating in air without degradation while being rolled to a radius of as small as ~200 μm. Flexible OFETs on Mylar substrates In this study, we use an OFET architecture that allows a very simple fabrication of self-supported OFETs with improved mechanical flexibility. Commercially available, ultra-thin, free-standing, insulating polymer membranes (2.5-μm-thick Mylar) are used in these OFETs as a substrate and a gate insulator at the same time. Metal gate, source and drain electrodes are pre-deposited on either sides of the membrane, followed by drop-casting solution-processable organic semiconductors, bis-(triisopropylsilylethynyl) pentacene (TIPS-pentacene) or bis-triethylsilylethynyl anthradithiophene (TES-ADT), between the source and drain electrodes ( Fig. 1 ). The semiconductor deposition, device wiring, handling and the mechanical bending tests have been performed in a normal laboratory environment (in air, under illumination, not in a clean room); all the electrical measurements have been performed in air as well. We found that highly crystalline films of both materials can be formed on Mylar substrates without any pre- or post-deposition treatments, such as a self-assembled monolayer growth or a solvent vapour annealing, typically necessary for crystallization on Si/SiO 2 wafers [11] . TIPS-pentacene and TES-ADT OFETs fabricated in this simple process exhibit characteristics indicative of correctly functioning high-performance field-effect transistors with very good linearity in the accumulation and saturation regimes and a charge carrier mobility in the range μ =0.1–0.4 cm 2 V −1 s −1 , comparable to the optimized devices reproducibly obtained on high-quality Si/SiO 2 wafers [11] , [12] . More importantly, we find that these OFETs exhibit an unprecedented electro-mechanical robustness in air, even when they are not encapsulated in any protective capping layer: their performance does not deteriorate after multiple bending of the accumulation channel to a radius as small as ~200 μm. Below, we first describe characterization and performance of our TIPS-pentacene OFETs, followed by the TES-ADT devices and finally we present the experimental investigation of the effect of mechanical strain (flexibility) on charge carrier mobility in these transistors. 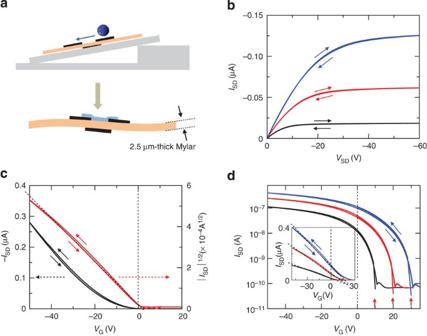Figure 1: Fabrication and transistor characteristics of flexible solution-processed TIPS-pentacene OFETs. (a) The semiconductor solution (blue sphere) is drop-cast on an ultra-thin Mylar sheet with pre-deposited gate, source and drain contacts, placed on a tilted glass slide. (b) The output characteristics of the resultant free-standing TIPS-pentacene OFET recorded atVG=−10 V (black), −20 V (red) and −30 V (blue). (c) The saturation-regime measurements:ISD(VG) andISD1/2(VG) recorded atVSD=−50 V; saturation mobility is 0.14 cm2V−1s−1. (d) The linear-regime measurements: transfer characteristicsISD(VG) of the same device recorded atVSD=10, 20 and 30 V (black, red and blue curves, respectively); linear mobility is 0.13 cm2V−1s−1. The vertical arrows indicate the field-effect onset. The inset shows the same data on a linear plot. Figure 1: Fabrication and transistor characteristics of flexible solution-processed TIPS-pentacene OFETs. ( a ) The semiconductor solution (blue sphere) is drop-cast on an ultra-thin Mylar sheet with pre-deposited gate, source and drain contacts, placed on a tilted glass slide. ( b ) The output characteristics of the resultant free-standing TIPS-pentacene OFET recorded at V G =−10 V (black), −20 V (red) and −30 V (blue). ( c ) The saturation-regime measurements: I SD ( V G ) and I SD 1/2 ( V G ) recorded at V SD =−50 V; saturation mobility is 0.14 cm 2 V −1 s −1 . ( d ) The linear-regime measurements: transfer characteristics I SD ( V G ) of the same device recorded at V SD =10, 20 and 30 V (black, red and blue curves, respectively); linear mobility is 0.13 cm 2 V −1 s −1 . The vertical arrows indicate the field-effect onset. The inset shows the same data on a linear plot. Full size image Ultra-flexible TIPS-pentacene OFETs Our previous study showed that ultra-thin Mylar membranes, vacuum laminated on the surface of organic single crystals, produce high-performance OFETs with conventional transistor characteristics, including high linear and saturation mobilities, nearly zero threshold voltage and negligible hysteresis [13] . Atomic force microscopy measurements reveal that the average surface roughness of these Mylar sheets is 0.7 nm (see Supplementary Fig. S1 ), comparable to high-quality SiO 2 wafers, establishing the basis for the use of these membranes as a gate dielectric in OFETs. Figure 1a depicts the method of solution-processed flexible OFET fabrication. First, silver gate and source-drain electrodes are evaporated on the opposite sides of the Mylar membrane through a shadow mask, so that the membrane serves not only as an ultra-thin substrate but also as a gate insulator. Second, the membrane is placed on an inclined support (a tilted glass slide) with the source and drain contacts facing up, and a solution of TIPS-pentacene in toluene is drop cast at the surface of the source-drain contacts using a micropipette. The support structure is only used during the solution deposition to help the droplet roll slowly from contact to contact, thus promoting the formation of crystalline TIPS-pentacene domains oriented along the channel. In the case of TES-ADT OFETs, a horizontal support surface was used (detailed optimized procedures for the growth of highly crystalline TIPS-pentacene and TES-ADT films on Mylar can be found in Methods). Figure 1b–d shows the performance of free-standing TIPS-pentacene OFETs on Mylar recorded in air: the devices exhibit nice characteristics both in the linear and saturation regimes, with negligible contact effects, nearly zero threshold voltage, small hysteresis and matching values of the linear and saturation mobility. Figure 1b shows that the output characteristics, I SD ( V SD ), are linear at small V SD , with a clear saturation of the source-drain current beyond the pinch-off point. Figure 1c shows the device performance in a saturation regime, in which the carrier density distribution between the source and drain contacts is non-uniform, with a pinch off of the accumulation channel near one of the contacts. It is important to note that our devices exhibit a linear I SD 1/2 ( V G ) dependence (solid red curve) in this regime, which confirms that the devices operate correctly, as expected from an ideal FET [14] . The field-effect mobility in the saturation regime, μ sat , has been calculated using the expression: I SD =[ W (2 L ) −1 ] μ sat C i ·( V G − V T ) [2] . The average mobility among 11 TIPS-pentacene devices was μ sat =0.15 cm 2 V −1 s −1 . Such result is very encouraging in light of the very simple fabrication process on cheap plastic foils used here. The transfer characteristics, I SD ( V G ), are shown in Fig. 1d (positive potential is applied to the source with respect to the grounded drain), demonstrating that the channel conductivity shows a strong field-effect modulation, with the field-effect onset voltage matching the applied positive V SD (indicated by vertical arrows). Such behaviour in OFETs is a manifestation of a negligible threshold voltage and thus negligible deep trap density in the accumulation channel [15] . The linear mobility, μ lin , was calculated from the linear transfer characteristics (inset in Fig. 1d ) according to the formula: μ lin =( LW −1 C i −1 V SD −1 )·( dI SD / dV G ). The average value among 15 TIPS-pentacene devices was μ lin =0.13 cm 2 V −1 s −1 (see Supplementary Fig. S2 ). The devices show nearly identical linear and saturation mobility values, as expected in correctly operating OFETs with negligible contact effects. The transfer curves are fairly linear (inset, Fig. 1d ), indicating that the carrier mobility in the accumulation regime is independent of the carrier density. This property is one of the most important prerequisites for applicability of the FET equations above commonly used for mobility calculations. In addition, μ lin does not depend on the source-drain voltage (see Supplementary Fig. S3 ), which is another sign of negligible contact resistance. To promote the growth of organic films with a well-defined crystalline orientation, various approaches have been suggested in the literature, including a liquid-sustaining blade held or moved along the Si/SiO 2 wafer [16] , or drop casting a semiconductor solution on an inclined Si/SiO 2 wafer [17] . These methods provide a driving force for oriented film growth. As mentioned above, our films have been grown by drop casting a semiconductor solution on an inclined Mylar surface, resulting in highly textured TIPS-pentacene films composed of striped crystalline domains with a preferential orientation along the direction of the inclination. To confirm that these domains actually carry the gate-induced current and are thus responsible for the high quality of our OFETs, we have investigated the correlation between the film texture orientation and the field-effect mobility ( Fig. 2 ). Here, θ is an angle between the long axis of the striped domains and the edges of the contacts that define the physical width of the accumulation channel, W ; θ can be easily controlled by changing the orientation of the Mylar sheet during drop-casting TIPS-pentacene solution. We have observed a systematic increase of the mobility when θ increases from 0 to 90°, with the maximum in μ reached for the striped domains propagating along the OFET channel ( θ =90°), as shown in Fig. 2 . The ratio of the field-effect mobility measured along the striped domains and perpendicular to them is ~15, consistent with the highly oriented texture of these films. This result agrees well with the anisotropy of approximately ten previously observed in oriented TIPS-pentacene films on Si/SiO 2 (ref. 12 ). It has to be emphasized that such an anisotropy should not be confused with the intrinsic anisotropy of the charge transport in organic crystals due to the anisotropic nature of transfer integrals in van der Waals molecular crystals [18] . In the OFETs based on single crystals of rubrene, tetracene and pentacene, the anisotropy of intrinsic mobility is typically in the range 3–5 (refs 19 , 20 , 21 , 22 ). The much greater apparent anisotropy observed in solution-grown polycrystalline films is due to highly oriented texture of these films, and thus it is a useful parameter for morphological characterization of these films [12] , [17] . 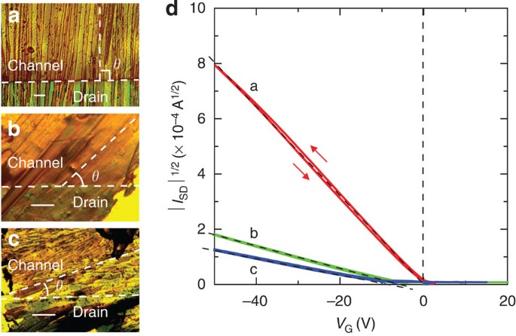Figure 2: Crystalline texture orientation and the electric field effect in TIPS-pentacene films grown on flexible Mylar sheets. (a–c) Optical microphotographs of the channel area in three OFETs with different orientation of the striped crystalline TIPS-pentacene domains with respect to the channel. The angle,θ, between the domain orientation and the contact edges is 90° ina, 42° inband 18° inc. Scale bars, 50 μm. (d) The saturation-regime characteristics,ISD1/2(VG), of the corresponding OFETs yield the saturation mobilities,μsat=0.2, 0.06 and 0.01 cm2V−1s−1fora–c, respectively. A clear correlation between the field-effect mobility and the film texture orientation is observed. Figure 2: Crystalline texture orientation and the electric field effect in TIPS-pentacene films grown on flexible Mylar sheets. ( a – c ) Optical microphotographs of the channel area in three OFETs with different orientation of the striped crystalline TIPS-pentacene domains with respect to the channel. The angle, θ , between the domain orientation and the contact edges is 90° in a , 42° in b and 18° in c . Scale bars, 50 μm. ( d ) The saturation-regime characteristics, I SD 1/2 ( V G ), of the corresponding OFETs yield the saturation mobilities, μ sat =0.2, 0.06 and 0.01 cm 2 V −1 s −1 for a – c , respectively. A clear correlation between the field-effect mobility and the film texture orientation is observed. Full size image Ultra-flexible TES-ADT OFETs We used a similar approach, drop casting on Mylar, to create TES-ADT OFETs with excellent electrical and mechanical characteristics. In this case, we found that using a highly concentrated solution (8 wt% TES-ADT in toluene), drop cast on a horizontally supported Mylar, is critical for obtaining thin, uniform and highly crystalline TES-ADT films with a very large domain size (up to ~0.5 mm) without any post-deposition treatments (for details, see Methods ). In this case, nucleation and growth of purple crystalline domains in the pink amorphous matrix can be clearly seen under an optical microscope in situ , as the solvent evaporates. These crystalline domains can quickly grow in size, eventually covering the entire surface of Mylar between the source and drain contacts with only a few grain boundaries (for movie of real-time crystallization of TES-ADT on Mylar see Supplementary Movie 1 ). These domains can be clearly discerned under a polarized optical microscope due to the contrast inversion that occurs when the polarizer angle is varied as shown in Fig. 3b . 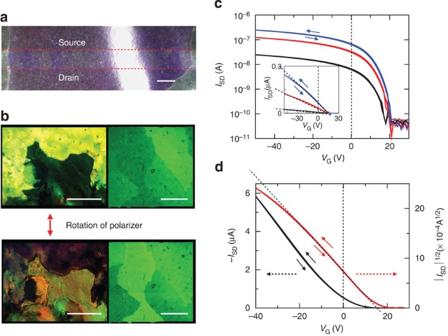Figure 3: Flexible solution-grown TES-ADT OFETs and their electrical characteristics. (a) Photograph of a TES-ADT OFET fabricated by drop casting on Mylar (scale bar, 500 μm). (b) Microphotographs of the channel area obtained in polarized optical microscope, showing large (few hundred μm in size) crystalline TES-ADT domains: a clear contrast inversion is observed when the polarizer is rotated (scale bars, 200 μm). (c) The linear-regime OFET measurements: semi-log plot of the transfer characteristics,ISD(VG), recorded atVSD=0.1 V (black), 0.5 V (red) and 1 V (blue). The inset shows the same data on a linear plot. (d) The saturation-regime OFET measurements:ISD(VG) andISD1/2(VG) characteristics recorded atVSD=−40 V.μlin≈μsat=0.38–0.4 cm2V−1s−1. Figure 3c shows the characteristics of the resultant TES-ADT OFETs in the linear and saturation regimes (measured in air, in the dark). Again, we find that the devices exhibit conventional FET behaviour with almost linear I SD ( V G ) and I SD 1/2 ( V G ) characteristics in the linear and saturation regimes, respectively, a high field-effect mobility ( μ lin ≈ μ sat =0.38–0.4 cm 2 V −1 s −1 ) and extremely small hysteresis. A slight nonlinearity of the transfer characteristics in these OFETs observed at high negative V G is likely related to an enhanced interfacial polaron scattering, when the thickness of the accumulation layer is reduced, as explained by the model developed by Mottaghi and Horowitz [23] . The output characteristics, I SD ( V SD ), show clear saturation of the current due to the channel pinch off (see Supplementary Fig. S4 ). It is worth noting that typical mobilities in solution-processed TES-ADT OFETs on Si/SiO 2 reported in the literature are 0.1–0.2 cm 2 V −1 s −1 , with Lee et al . [11] , [24] recently reporting enhanced mobility of up to 0.4 cm 2 V −1 s −1 achieved by optimization of solvent vapour annealing. This indicates that performance of our OFETs is comparable to some of the best devices grown on Si/SiO 2 substrates. The combination of high performance, mechanical flexibility (see below) and a very simple fabrication route highlights the unique and highly desirable characteristics of this approach. Figure 3: Flexible solution-grown TES-ADT OFETs and their electrical characteristics. ( a ) Photograph of a TES-ADT OFET fabricated by drop casting on Mylar (scale bar, 500 μm). ( b ) Microphotographs of the channel area obtained in polarized optical microscope, showing large (few hundred μm in size) crystalline TES-ADT domains: a clear contrast inversion is observed when the polarizer is rotated (scale bars, 200 μm). ( c ) The linear-regime OFET measurements: semi-log plot of the transfer characteristics, I SD ( V G ), recorded at V SD =0.1 V (black), 0.5 V (red) and 1 V (blue). The inset shows the same data on a linear plot. ( d ) The saturation-regime OFET measurements: I SD ( V G ) and I SD 1/2 ( V G ) characteristics recorded at V SD =−40 V. μ lin ≈ μ sat =0.38–0.4 cm 2 V −1 s −1 . Full size image Mechanical robustness of the solution-processed OFETs We have performed extensive tests of the mechanical flexibility of our free-standing TIPS-pentacene and TES-ADT OFETs to investigate the degree of their electrical stability on bending. 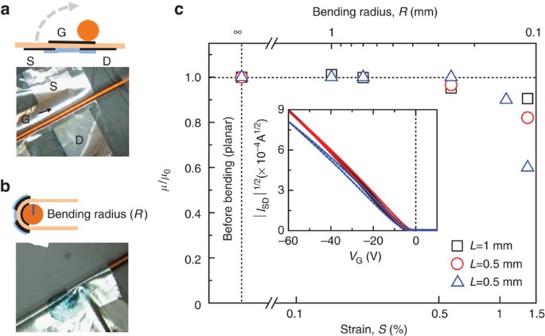Figure 4: Test of electro-mechanical stability of solution-processed OFETs before and after bending. (a,b) Schematics of the bending test and photographs of OFETs in a planar and bent configurations. The devices were bent around a tightly drawn varnish-coated copper wire (orange) of varied radius,R, with the semiconducting film (blue) facing outwards. (c) The dependence of the field-effect mobility on the bending radius and the applied strain (μis normalized to the mobility,μ0, in as-prepared devices). The bending results are shown for three different OFETs with channel lengths 0.5 and 1 mm measured in the planar configuration before and after ten bending cycles for eachR. The inset shows an example of the saturation-regime characteristics,ISD1/2(VG), obtained atVSD=−60 V for as-prepared OFET (black), the same device after ten bending toR=260 μm (red) and another ten bending cycles toR=110 μm (blue). These measurements of un-encapsulated OFETs have been carried out in air. Figure 4 shows the electrical performance of the OFETs tested in a planar (flattened out) geometry before and after multiple bending stresses; Fig. 5 shows another type of test—measurements performed during bending (in a stressed configuration). These bending tests have been performed in air, under indoor illumination. The gate leakage current was monitored in each measurement before, after and during bending; it did not exceed a few hundred pA (see Supplementary Fig. S5 ). In the first type of test, as-prepared OFETs with different channel lengths have been initially characterized in a planar geometry, and then the devices were bent multiple times (ten times for each radius) against a varnish-coated copper wire of varied radius, R , as shown in Fig. 4a , and finally measured again in a planar geometry. The wire was carefully positioned in the channel between the source and drain contacts, so that the bending-induced strain was applied to the semiconducting channel of the OFETs. Figure 4c shows the mobility as a function of the bending radius measured in three different OFETs. The mobility is normalized to the initial value in the devices before the bending test. As an example, the inset in Fig. 4c shows a few saturation-regime characteristics, I SD 1/2 ( V G ), obtained before and after ten bending stresses to the radius as small as 110 μm. Remarkably, these unencapsulated OFETs operate without significant degradation after bending to a radius as small as 260 μm. This is about one order of magnitude smaller than the smallest bending radius reported for OFETs without encapsulation. Both the TIPS-pentacene and TES-ADT transistors gave similar results in this type of bending test. Figure 4: Test of electro-mechanical stability of solution-processed OFETs before and after bending. ( a , b ) Schematics of the bending test and photographs of OFETs in a planar and bent configurations. The devices were bent around a tightly drawn varnish-coated copper wire (orange) of varied radius, R , with the semiconducting film (blue) facing outwards. ( c ) The dependence of the field-effect mobility on the bending radius and the applied strain ( μ is normalized to the mobility, μ 0 , in as-prepared devices). The bending results are shown for three different OFETs with channel lengths 0.5 and 1 mm measured in the planar configuration before and after ten bending cycles for each R . The inset shows an example of the saturation-regime characteristics, I SD 1/2 ( V G ), obtained at V SD =−60 V for as-prepared OFET (black), the same device after ten bending to R =260 μm (red) and another ten bending cycles to R =110 μm (blue). These measurements of un-encapsulated OFETs have been carried out in air. 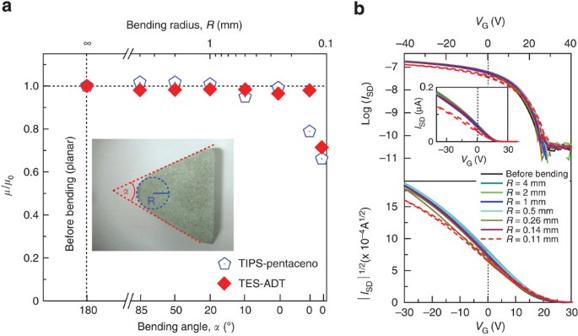Figure 5: Test of electro-mechanical stability of solution-processed OFETs during bending. (a) Dependence of the normalized mobility on the bending radius,R, and bending angle,α(open pentagons: TIPS-pentacene, solid rhombs: TES-ADT).Randαare defined by the shape of the wedge-like support structures, against which the OFETs are bent (inset).α=180° corresponds to a flat (planar) OFET geometry, andα=0 corresponds to an OFET wrapped around a half circle. The measurements have been carried out with the devices in a bent configuration (under strain), in air, under laboratory illumination. (b) An example of the transfer characteristics of a TES-ADT OFET in the linear regime atVSD=1 V (upper panel) and saturation regime atVSD=−30 V (lower panel) recorded during bending of the device to various radii. Full size image Figure 5: Test of electro-mechanical stability of solution-processed OFETs during bending. ( a ) Dependence of the normalized mobility on the bending radius, R , and bending angle, α (open pentagons: TIPS-pentacene, solid rhombs: TES-ADT). R and α are defined by the shape of the wedge-like support structures, against which the OFETs are bent (inset). α =180° corresponds to a flat (planar) OFET geometry, and α =0 corresponds to an OFET wrapped around a half circle. The measurements have been carried out with the devices in a bent configuration (under strain), in air, under laboratory illumination. ( b ) An example of the transfer characteristics of a TES-ADT OFET in the linear regime at V SD =1 V (upper panel) and saturation regime at V SD =−30 V (lower panel) recorded during bending of the device to various radii. Full size image Figure 5 shows the second type of bending test, in which the OFETs were bent against specially designed wedge-like structures, and their electrical characteristics were recorded in situ in the bent configuration. The shape of the wedge-like structure defines the bending radius ( R ) of the OFET channel and the angle ( α ) between it’s sides, as shown in the inset in Fig. 5 : α =180° corresponds to a planar OFET configuration, whereas α =0 corresponds to an OFET bent around half of the circumference. Figure 5a shows the normalized mobility of these devices under strain as a function of the bending radius and angle. Figure 5b shows an example of transfer characteristics of a TES-ADT OFET in the linear and saturation regimes recorded during this bending test. These data show that the transistors perform very well not only after bending but also while the strain is applied to the semiconducting channel. The critical bending radius of these unencapsulated OFETs is extremely small (~200 μm) and consistent in both types of the bending tests ( Figs 4 and 5 ). In addition to the measurements under tensile strain, we have also performed measurements of these OFETs under a compressive strain with sequentially decreasing bending radius and angle by using a similar method as in Fig. 5 . We have not observed any significant deterioration of the field-effect mobility until the bending radius reached 260 μm (see Supplementary Fig. S6 ). This indicates that electro-mechanical stability of these solution-processed organic semiconductors under tensile and compressive strains is similar. Our study reveals that large-grain crystalline organic semiconductors grown from solutions into thin solid films exhibit a substantial mechanical flexibility without deterioration of their good electrical transport properties. The field-effect mobility in both TIPS-pentacene and TES-ADT remains largely unaffected by bending to a radius as small as ~200 μm (~1% strain). The self-supported architecture of these devices that takes advantage of ultra-thin polymer membranes as substrates results in extremely small total device thickness of 2.5 μm. This helps to perform basic electro-mechanical studies (flexibility) of these electronic materials and access the regime of extreme bending. Indeed, the strain, S , induced in a thin film supported by a flexible substrate is related to the substrate thickness as: S ≈0.5 ( t sub + t film )· R −1 , where t sub and t film are the thicknesses of the substrate and the film, respectively [25] . In our case, the thickness of the organic semiconductor film is 30–40 nm. Thus, using a 2.5-μm-thick Mylar membrane as a gate insulator and a substrate simultaneously allows to markedly reduce the strain exerted on the semiconducting channel (max· S ≈0.8%), even when the OFETs are wrapped around objects with extremely small radii ~200 μm. The results of this study are different from the recent studies of OFETs on plastic substrates in several critical aspects. First, we have investigated solution-processed crystalline organic semiconductors based on small organic molecules, for which rigorous tests of mechanical flexibility were lacking. Compared with conjugated polymers [9] , [10] , these materials have an advantage of higher purity, molecular monodispersity, crystallinity, as well as typically greater linear charge carrier mobilities. They also compare favourably to organic semiconductors evaporated in high vacuum in terms of the fabrication cost and possibility of integration with printed electronics. Second, we use a device architecture, in which the entire device itself is a substrate, resulting in ultra-thin flexible OFETs that allow performing extensive basic studies of the impact of strain on electronic properties of these semiconductors. Even though such an approach is far from being optimized for real applications, it is a very useful tool for fundamental studies of electro-mechanical properties. Our experiment also shows that for such thin devices it is not necessary to place the transistor in a neutral strain position by capping it with an extra insulating layer. Third, we have performed rigorous electro-mechanical measurements in a variety of stress configurations and geometries, all of which gave consistent results. In conclusion, we used a very simple method for fabrication of high-performance small-molecule OFETs by drop-casting solution-processed organic semiconductors on inexpensive ultra-thin plastic membranes, resulting in devices that exhibit extreme mechanical flexibility without degradation of their electrical performance. These few micrometre thick devices can be rolled multiple times to a radius of ~200 μm and still function normally. The charge carrier mobility of 0.1–0.4 cm 2 V −1 s −1 in these flexible TIPS-pentacene and TES-ADT OFETs is comparable to the best reproducible values obtained in these materials using expensive rigid Si/SiO 2 wafers. This basic study of electro-mechanical properties of OFETs demonstrates a potential of solution-grown crystalline organic semiconductors for applications in low-cost, flexible, plastic electronics. Materials TIPS-pentacene and TES-ADT were synthesized following previously published procedures [26] , [27] . The synthesized materials have been purified by multiple solvent recrystallization from acetone (TIPS-pentacene) or hexane (TES-ADT) [28] . Device fabrication Commercially available free-standing Mylar membranes (2.5-μm-thick polyethylene terephthalate sheets with C i =1.14 nF cm −2 , purchased from Chemplex) served as a substrate and a gate insulator. Both gate electrode and the source-drain contacts are deposited by thermal evaporation of silver through a shadow mask on the opposite sides of the Mylar sheet by first evaporating the gate electrode on one side of the insulating membrane, then rotating the sample holder in situ (without breaking the vacuum) by 180° and evaporating the source-drain contacts on the other side. Such a structure based on a thin plastic film has been suggested before for vacuum-evaporated pentacene thin-film transistors, in which the device parameters (mobility and threshold voltage) depended strongly on mechanical flexing, thus suggesting a promising application in pressure sensors [28] . Typical channel dimensions defined by the shadow masks in our devices were as follows: L =500 or 1,000 μm and W =4–6 mm. Minimization of the channel dimensions to micro scale is possible by using evaporation through a shadow mask that defines a short channel or photolithography. In the case of TES-ADT, a brief ultraviolet-ozone treatment of the Mylar with pre-deposited Ag contacts helps to form more uniform and very thin TES-ADT film over a large area. Freshly prepared 5 wt% solution of TIPS-pentacene and 8 wt% solution of TES-ADT in toluene (Fisher Scientific, CAS 108-88-3) were used. The semiconductor solution was drop-cast using a micropipette (1 μl per device) onto the surface of Mylar sheets with pre-deposited contacts. We used Molecular Bioproduct ART (Aerosol Resistant) or BIO-CERT high-purity plastic micropipette tips. In the case of TIPS-pentacene, to enhance the film crystallinity and promote an oriented domain growth, the Mylar membrane was placed on an inclined support structure. In the case of TES-ADT, inclination did not result in oriented domains, and hence all consecutive devices were fabricated by drop-casting solution on a horizontal substrate. After solvent evaporation and formation of crystalline films, the Mylar sheets were peeled off the supporting glass slide and used as free-standing flexible OFETs. As contact leads, we used a 25-μm-thick gold wire attached to the silver source and drain contact pads with a conductive silver paint. Electrical characterization of devices All measurements reported here have been performed at room temperature, in air. Keithley Source-Meters K-2400 and Electrometers K-6514 were used for FET measurements. Typical rate of gate voltage and source-drain voltage sweeps in our I SD ( V G ) and I SD ( V SD ) measurements is 1–2 V s −1 . Tests of mechanical flexibility (bending) In the first type of bending test ( Fig. 4 ), tightly drawn straight pieces of varnish-coated copper wire with radii R =1, 0.7, 0.26, 0.14 and 0.11 mm were used. The OFETs were bent around the wire ten times with the (unencapsulated) organic semiconductor film facing outwards (tensile strain). The OFET measurements were performed in a planar configuration before and after ten bending stresses. For measurements in a compressive strain regime, see the Supplementary Information . In the second type of bending test ( Fig. 5 ), rigid ceramic wedge-like support structures have been used. Each wedge is characterized by a certain curvature and angle between the sides that define the bending radius, R , and angle, α , respectively. The devices have been first measured in a planar configuration and then again while bent around the wedges. All mechanical bending tests have been performed in air under indoor illumination. How to cite this article: Yi, H.T. et al . Ultra-flexible solution-processed organic field-effect transistors. Nat. Commun. 3:1259 doi: 10.1038/ncomms2263 (2012).